Auxin-Binding Protein 1 is a negative regulator of the SCFTIR1/AFBpathway Auxin is a major plant hormone that controls most aspects of plant growth and development. Auxin is perceived by two distinct classes of receptors: transport inhibitor response 1 (TIR1, or auxin-related F-box (AFB)) and auxin/indole-3-acetic acid (AUX/IAA) coreceptors, that control transcriptional responses to auxin, and the auxin-binding protein 1 (ABP1), that controls a wide variety of growth and developmental processes. To date, the mode of action of ABP1 is still poorly understood and its functional interaction with TIR1/AFB–AUX/IAA coreceptors remains elusive. Here we combine genetic and biochemical approaches to gain insight into the integration of these two pathways. We find that ABP1 is genetically upstream of TIR1/AFBs; ABP1 knockdown leads to an enhanced degradation of AUX/IAA repressors, independently of its effects on endocytosis, through the SCF TIR1/AFB E3 ubiquitin ligase pathway. Combining positive and negative regulation of SCF ubiquitin-dependent pathways might be a common mechanism conferring tight control of hormone-mediated responses. Among the plant hormones that control plant growth and development, auxin has been implicated in virtually every aspect. This predominant role of auxin relies on its critical involvement in the regulation and coordination of cell division, cell expansion and differentiation that sustain growth, initiation and formation of new organs or adaptive responses to environmental stimuli [1] , [2] . Within the last decade, molecular and genetic evidence established the importance of auxin-mediated transcriptional responses involving the auxin coreceptors transport inhibitor response 1/auxin-related F-box proteins (TIR1/AFB) and auxin/indole-3-acetic acid (AUX/IAA) repressors [3] , [4] . Auxin favours AUX/IAA recruitment by TIR1/AFBs within SCF TIR1/AFB ubiquitin ligase E3 complexes that promotes their polyubiquitination and degradation through the ubiquitin/26S proteasome system (UPS) [3] , [5] . AUX/IAAs are transcriptional repressors limiting in time and space the transcription of auxin-responsive genes; their degradation is a prerequisite for modification of gene expression. Various developmental defects were reported for gain-of-function aux/iaa mutants expressing stable AUX/IAA proteins, thus disturbing a broad range of auxin-mediated responses [6] . Surprisingly, little is known of the effects resulting from loss of function of AUX/IAA repressors, potentially because of significant redundancy within the gene family [7] , [8] . Loss of function of up to four TIR1/AFB proteins leads to three different phenotypes ranging from rootless seedlings (group I) to nearly normal ones (group III) [9] . In addition to TIR1/AFB–AUX/IAA coreceptors, auxin is also perceived by ABP1 that is associated with the plasma membrane and was shown to be involved in the regulation of ion fluxes at the plasma membrane [10] and, more recently, in the activation of ROP GTPases [11] , [12] in response to auxin. ABP1 was also shown to be essential for clathrin-dependent endocytosis, acting as a positive factor for clathrin recruitment to the plasma membrane and inhibiting this process after binding to auxin [11] , [13] . The contribution of these early and potentially transient responses to growth and development is however still unknown. Loss of function of ABP1 and post-embryonic functional inactivation of the protein by inducible cellular immunization or antisense were demonstrated to provoke lethality and severe developmental defects at all stages of development [14] , [15] , [16] . At the cellular level, ABP1 was shown to be required for cell division [14] , [16] , [17] and also for cell expansion in shoot tissues [14] , [15] , [16] , [18] . Interestingly, ABP1 was also reported to be required for a tight regulation of a number of auxin response genes [16] , thus suggesting that ABP1 and TIR1/AFB–AUX/IAA collectively contribute to mediate auxin responses. Here, to further investigate the molecular mechanism by which ABP1 controls root growth, we have studied the relationship between ABP1 and TIR1/AFB pathways. We report that most developmental defects observed after ABP1 knockdown result from transcriptional alterations and that regulation of AUX/IAA homeostasis requires ABP1. ABP1 promotes AUX/IAA stability independently from its action on endocytosis. We conclude that ABP1 behaves as a negative regulator of the SCF TIR1/AFB signalling pathway and that transcriptional regulation results from a critical balance between these two pathways. TIR1/AFB are epistatic to ABP1 To gain insight into the understanding of the cross-talk between ABP1 and TIR1/AFB pathways, we investigated genetic interactions between both pathways. We focused on the analysis of homozygous lines for ABP1 knockdown (SS12K9) in single, double and triple tir1-1afb2-1afb3-1 mutants. Inactivation of ABP1 in single mutants led to plants exhibiting typical ABP1 knockdown root phenotypes as illustrated for tir1-1 ( Fig. 1a ). However, inactivation of ABP1 in various double mutants and in the triple tir1-1afb2-1afb3-1 mutant led to a striking result. Depending on the combination of mutants, phenotypes associated with the inactivation of ABP1 were either reduced as observed for tir1-1afb3-1 and afb2-1afb3-1 double mutants ( Fig. 1b ), or completely vanished for tir1-1afb2-1 mutant and the triple mutant ( Fig. 1a ). The differential effect of double mutations confirms predominance of TIR1 and AFB2 in roots [19] ; however, AFB3 is also clearly involved. Conversely, post-embryonic ABP1 knockdown had no effect on the variability of phenotypes reported for the triple tir1-1afb2-1afb3-1 mutant [9] but the typical long wavy primary root phenotype resulting from group III triple tir/afb mutations was observed ( Fig. 1a ). Importantly, we confirmed that the scFv12 antibody responsible for the inactivation of ABP1 was properly induced and produced in response to ethanol induction in the triple mutant background ( Fig. 1c ). In addition, growth inhibition resulting from ABP1 inactivation was recovered in SS12K9, tir1-1afb2-1afb3-1 plants backcrossed with Col0, (thus, heterozygous for all mutations and for the scFv12 construct), demonstrating that the scFv12 was still fully efficient in these plants ( Fig. 1d ). These genetic analyses confirm the partial redundancy between TIR1, AFB2 and AFB3, and more importantly reveal that TIR1/AFBs are epistatic to ABP1 . 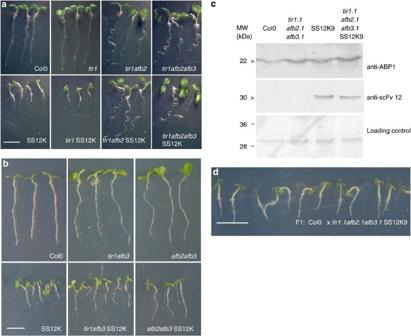Figure 1: Genetic relationship between TIR1/AFBs and ABP1. (a) Phenotypes of 4-day-old seedlings oftir1-1, doubletir1-1,afb2-1and tripletir1-1,afb2-1,afb3-1mutants and SS12K9 into these mutant backgrounds mediating functional inactivation of ABP1; all induced by ethanol since germination. Col0 and SS12K phenotypes are included for comparison. (b) Phenotypes of 4-day-old seedlings ofafb2-1afb3-1andtir1-1afb3-1double mutants and SS12K9 into these mutant backgrounds mediating functional inactivation of ABP1; all induced by ethanol since germination. (c) ABP1 and scFv12 recombinant antibodies were detected by western blot using mAb34 anti-ABP1 monoclonal antibody and anti-scFv E-Tag antibodies, respectively. Full image of blots are shown as aSupplementary Fig. S1. (d) Phenotype of ethanol-induced seedlings resulting from the backcross of homozygous plants for SS12K9,tir1-1afb2-1afb3-1with WT Col0. F1 plants are heterozygous for all mutations and for the ethanol-inducible construct responsible for ABP1 inactivation. Scale bars, 5 mm (a,b,d). Figure 1: Genetic relationship between TIR1/AFBs and ABP1. ( a ) Phenotypes of 4-day-old seedlings of tir1-1 , double tir1-1 , afb2-1 and triple tir1-1 , afb2-1 , afb3-1 mutants and SS12K9 into these mutant backgrounds mediating functional inactivation of ABP1; all induced by ethanol since germination. Col0 and SS12K phenotypes are included for comparison. ( b ) Phenotypes of 4-day-old seedlings of afb2-1afb3-1 and tir1-1afb3-1 double mutants and SS12K9 into these mutant backgrounds mediating functional inactivation of ABP1; all induced by ethanol since germination. ( c ) ABP1 and scFv12 recombinant antibodies were detected by western blot using mAb34 anti-ABP1 monoclonal antibody and anti-scFv E-Tag antibodies, respectively. Full image of blots are shown as a Supplementary Fig. S1 . ( d ) Phenotype of ethanol-induced seedlings resulting from the backcross of homozygous plants for SS12K9, tir1-1afb2-1afb3-1 with WT Col0. F1 plants are heterozygous for all mutations and for the ethanol-inducible construct responsible for ABP1 inactivation. Scale bars, 5 mm ( a , b , d ). Full size image TIR1/AFB expression is not dependent on ABP1 To better understand the genetic relationship between ABP1 and TIR1/AFBs, we first investigated whether ABP1 affects TIR1 and AFB expression. We studied the accumulation of corresponding mRNAs in roots inactivated for various time for ABP1 ( Fig. 2a ). No difference was observed for TIR1 and AFB1 , and only a very subtle decrease of AFB2 and AFB3 mRNA was observed over time. Using immunodetection of the TIR1-HA reporter [20] , no significant change in TIR1 protein was observed in response to ABP1 inactivation, suggesting that ABP1 does not act through quantitative changes of TIR1 ( Fig. 2b ). We then investigated whether ABP1 directly affects the half-life of TIR1/AFB substrates. 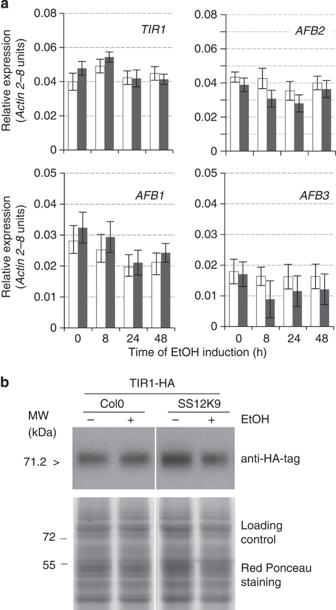Figure 2: Inactivation of ABP1 does not affect the expression ofTIR1andAFBs. (a) Quantitative RT–PCR analysis ofTIR1,AFB1,AFB2etAFB3in WT (in white) and SS12K9 (in grey) after various times of ethanol induction. All data were normalized with respect toACTIN2-8and expressed in equivalentACTINunits. Error bars are s.d.,n=6 (three biological replicates, each in two experimental repeats). (b) Immunodetection of TIR-HA reporter protein in Col0 and SS12K9 backgrounds, with or without inactivation of ABP1. Red ponceau staining is included as a loading control. Full image of blots are shown as aSupplementary Fig. S1. Figure 2: Inactivation of ABP1 does not affect the expression of TIR1 and AFBs . ( a ) Quantitative RT–PCR analysis of TIR1 , AFB1 , AFB2 et AFB3 in WT (in white) and SS12K9 (in grey) after various times of ethanol induction. All data were normalized with respect to ACTIN2-8 and expressed in equivalent ACTIN units. Error bars are s.d., n =6 (three biological replicates, each in two experimental repeats). ( b ) Immunodetection of TIR-HA reporter protein in Col0 and SS12K9 backgrounds, with or without inactivation of ABP1. Red ponceau staining is included as a loading control. Full image of blots are shown as a Supplementary Fig. S1 . Full size image ABP1 controls AUX/IAA stability Next we studied the half-life of the well-described heat-shock (HS)-inducible AXR3NT-GUS reporter, which was initially used to demonstrate that AUX/IAAs are short-lived nuclear proteins [21] , in the context of ABP1 inactivation. Two constructs were introgressed into the SS12K9 conditional ABP1 line [5] : the pHS:AXR3NT-GUS reporter and the same construct containing a point mutation within the degron of domain II pHS:axr3.1NT-GUS that impairs the interaction with TIR1 (ref. 21 ). To compare protein half-life from plant roots of similar development, 4-day-old seedlings of wild-type (WT) and SS12K9 reporter lines were grown in the absence of ethanol induction and were exposed overnight to ethanol vapour to induce inactivation of ABP1 in SS12K9 before a 3-h HS treatment on plates. Reporter abundance was estimated by β-glucuronidase (GUS) staining and GUS activity was quantified by fluorimetry on protein extracts of a large number of roots to average plant to plant differences ( Fig. 3 ). In WT extracts, the protein accumulated during the HS was slowly degraded, with an EC50 between 60 and 80 min ( Fig. 3b ), in accordance with previous reports [21] , [22] . Immediately after HS, only one third of the AXR3NT-GUS protein quantified in WT was measured in roots inactivated for ABP1 and GUS activity dropped to baseline within 10 min. The low level of protein reporter could result either from a decrease in biosynthesis or from increased degradation. Quantification of GUS activity in plants expressing pHS:axr3.1NT-GUS constructs revealed that neither the response to HS nor the capacity of protein biosynthesis were affected in SS12K9 ( Fig. 3d ). Mutated axr3.1NT-GUS proteins exhibited an elevated stability over time in both WT and ABP1-inactivated backgrounds ( Fig. 3d,e ). In the absence of functional ABP1, the axr3.1 single mutation in domain II is sufficient to avoid degradation, indicating that AUX/IAA enhanced degradation in SS12K9 relies on their interaction with TIR1/AFB F-box proteins as previously reported in WT background [21] . To verify that the low level of AXR3NT-GUS in SS12K9 resulted from an increased and proteasome-dependent degradation, HS induction was performed in the presence of the proteasome inhibitor MG132. In SS12K9, MG132 treatment restored the level of AXR3NT-GUS almost to that observed in WT in the absence of inhibitor ( Fig. 3c ), thus confirming that the observed differences came from an increased degradation of AXR3NT-GUS resulting from functional inactivation of ABP1. Interestingly, in WT, a slight increase in the amount of AXR3NT-GUS was also observed in the presence of MG132 during HS ( Fig. 3c ), suggesting that partial degradation of the reporter already takes place during HS treatment. The quantity of AXR3NT-GUS protein detected at the end of the HS results from an equilibrium between production and degradation. This equilibrium is severely shifted in favour of degradation when ABP1 is not functional, indicating that ABP1 behaves as a negative regulator of AUX/IAA degradation. 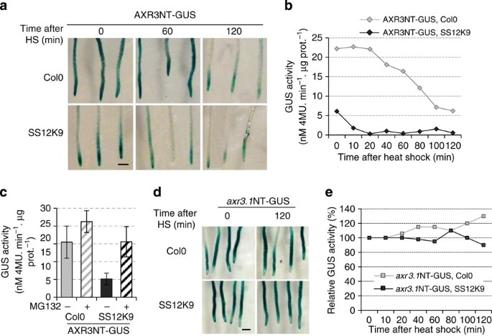Figure 3: ABP1 pathway stabilizes AUX/IAA repressors. (a) GUS staining in roots at various times after HS treatment of overnight ethanol-induced 4-day-old WT and SS12K9 seedlings expressing thepHS:AXR3NT-GUSconstruct. (b) Quantification and kinetic analyses of GUS activity in root samples as ina. Activity is expressed in 4-methylumbelliferone (MU) per minute and μg protein. (c) Quantification of GUS activity corresponding to accumulation of AXR3NT-GUS in overnight ethanol-induced roots treated or not with MG132 proteasome inhibitor during HS. Error bars represent s.d.,n=5 biological replicates. (d) GUS staining at various times after HS treatment in overnight ethanol-induced WT and SS12K9 roots expressing thepHS:axr3.1NT-GUSconstruct. (e) Quantification and kinetic analyses of GUS activity in root samples as ind. Scale bars, 500 μm (a,d). Figure 3: ABP1 pathway stabilizes AUX/IAA repressors. ( a ) GUS staining in roots at various times after HS treatment of overnight ethanol-induced 4-day-old WT and SS12K9 seedlings expressing the pHS:AXR3NT-GUS construct. ( b ) Quantification and kinetic analyses of GUS activity in root samples as in a . Activity is expressed in 4-methylumbelliferone (MU) per minute and μg protein. ( c ) Quantification of GUS activity corresponding to accumulation of AXR3NT-GUS in overnight ethanol-induced roots treated or not with MG132 proteasome inhibitor during HS. Error bars represent s.d., n =5 biological replicates. ( d ) GUS staining at various times after HS treatment in overnight ethanol-induced WT and SS12K9 roots expressing the pHS:axr3.1NT-GUS construct. ( e ) Quantification and kinetic analyses of GUS activity in root samples as in d . Scale bars, 500 μm ( a , d ). Full size image To address whether the suppression of ABP1 knockdown phenotypes by tir1/afb combined mutations results from a restoration of AUX/IAA stability, we analysed AXR3NT-GUS reporter in SS12K9, tir/afb mutants ( Fig. 4 ). Gus staining confirmed that AXR3NT-GUS accumulates after inactivation of ABP1 in the mutant background, indicating that suppression of the phenotype resulting from ABP1 inactivation by the tir/afb mutations is correlated with a restoration of endogenous AUX/IAA stability. These data reveal that primary root growth requires repression of auxin-mediated transcriptional responses and that ABP1 is required to maintain this repression via stabilization of AUX/IAA repressors. In other words, the ABP1-mediated pathway counteracts the TIR1/AFB–AUX/IAA pathway by increasing the stability of AUX/IAA repressors to control plant growth and development. 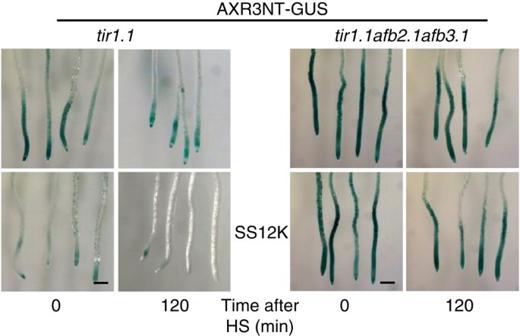Figure 4: Suppression of ABP1 knockdown phenotype correlates with stabilization of AUX/IAA. Four-day-old seedlings oftir1-1and tripletir1-1,afb2-1,afb3-1mutants with functional ABP1 or in SS12K9 were ethanol induced overnight before HS treatment. GUS staining detecting the accumulation of AXR3NT-GUS was performed at the end of the HS treatment or after 120 min. Scale bars, 500 μm. Figure 4: Suppression of ABP1 knockdown phenotype correlates with stabilization of AUX/IAA. Four-day-old seedlings of tir1-1 and triple tir1-1,afb2-1,afb3-1 mutants with functional ABP1 or in SS12K9 were ethanol induced overnight before HS treatment. GUS staining detecting the accumulation of AXR3NT-GUS was performed at the end of the HS treatment or after 120 min. Scale bars, 500 μm. Full size image ABP1 acts specifically on auxin-dependent targets The regulation of protein turnover through the UPS was shown to have critical roles in almost every aspect of plant growth and development, including modulation of phytohormone signalling [23] . Considering the severe phenotypes resulting from ABP1 inactivation as well as the lethality of the null Arabidopsis mutant [15] , we questioned whether the effect of ABP1 on protein stability resulted from a broad alteration of Skp, Cullin, F-box containing complex (SCF)-mediated protein degradation or was specific to SCF TIR1/AFBs E3 ubiquitin ligases targeting AUX/IAA repressors. We first investigated whether ABP1 affects one of the major mechanism modulating ubiquitin E3 ligases by analysing the effect of ABP1 inactivation on the steady-state level of modified SCF scaffold protein CULLIN1 (CUL1) by the ubiquitin-like RUB (related to ubiquitin [24] ). No significant change in the ratio of rubylated versus non-rubylated CUL1 was detected after the inactivation of ABP1 ( Fig. 5a ), suggesting that ABP1 is not acting on this mechanism. We then investigated whether ABP1 inactivation affects the stability of other well-known UPS-dependent regulatory proteins starting with JAZ repressors of the jasmonate pathway. The COI1 gene that triggers ubiquitination of JAZ is the closest gene to TIR1 and AFBs within the LRR subfamily of F-box proteins [9] , [19] . We analysed the effect of ABP1 inactivation on JAZ1-GUS protein half-life [25] . Inactivation of ABP1 had no significant impact on the turnover of JAZ proteins ( Fig. 5b ), indicating that inactivation of ABP1 does not affect a central mechanism shared by distinct SCF complexes. Finally, we studied the degradation of the growth-repressing DELLA proteins [26] , using the pRGA:RGA-GFP reporter [27] . RGA-GFP protein was degraded in both genotypes in response to gibberellic acid (GA3) treatment; however, GA-induced RGA-GFP degradation was delayed in ABP1-inactivated roots ( Fig. 5c ). Interestingly, this effect is reminiscent of the delay in GA-induced RGA degradation caused by auxin depletion in roots [27] . On the basis of these results, we propose that ABP1 inactivation promotes rather specifically AUX/IAA repressors for degradation. 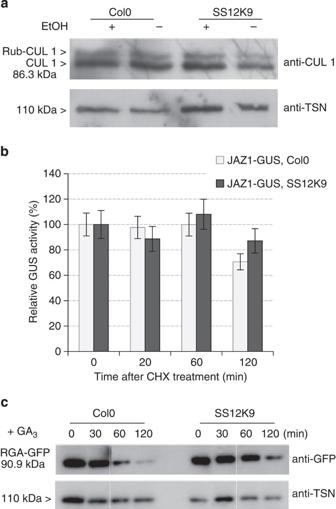Figure 5: ABP1 acts specifically on AUX/IAA substrates. (a) ABP1 does not affect the steady-state level of CUL1 modification. Rubylated and non-rubylated CUL1 in overnight ethanol-induced WT and SS12K9 root extracts were detected using anti-CUL1 antibodies. (b) ABP1 inactivation does not affect JAZ1 half-life. GUS activity resulting from the expression of the p35S:JAZ1-GUS reporter was measured in roots of overnight ethanol-induced WT (in white) and SS12K9 (in grey) treated for various times with cycloheximide. To evaluate the relative stability of JAZ1-GUS reporter as a possible effect of ABP1 inactivation, the experiment was performed without any JA exogenous treatment. Error bars are s.d.,n=3 biological replicates. (c) Inactivation of ABP1 delays degradation of RGA-GFP. Samples of overnight ethanol-induced seedlings were collected after treatment with 5 μM GA3 for the indicated time. RGA-GFP was detected by western blot using anti-GFP antibodies. Full image of blots inaandcare shown as aSupplementary Fig. S1. Figure 5: ABP1 acts specifically on AUX/IAA substrates. ( a ) ABP1 does not affect the steady-state level of CUL1 modification. Rubylated and non-rubylated CUL1 in overnight ethanol-induced WT and SS12K9 root extracts were detected using anti-CUL1 antibodies. ( b ) ABP1 inactivation does not affect JAZ1 half-life. GUS activity resulting from the expression of the p35S:JAZ1-GUS reporter was measured in roots of overnight ethanol-induced WT (in white) and SS12K9 (in grey) treated for various times with cycloheximide. To evaluate the relative stability of JAZ1-GUS reporter as a possible effect of ABP1 inactivation, the experiment was performed without any JA exogenous treatment. Error bars are s.d., n =3 biological replicates. ( c ) Inactivation of ABP1 delays degradation of RGA-GFP. Samples of overnight ethanol-induced seedlings were collected after treatment with 5 μM GA3 for the indicated time. RGA-GFP was detected by western blot using anti-GFP antibodies. Full image of blots in a and c are shown as a Supplementary Fig. S1 . Full size image ABP1 affects AUX/IAA stability independently from its effect on endocytosis On the basis of the current model of auxin-dependent transcriptional regulation, an increased degradation of AUX/IAA repressors might result either from an increase in auxin content promoting interaction of TIR1/AFBs and AUX/IAAs coreceptors, or from a modulation of AUX/IAA repressor half-life through differential interaction with TIR1/AFBs independently of the presence of auxin [28] . Several lines of evidence support that the inactivation of ABP1 does not result in an increase in auxin content that would be responsible for enhanced AUX/IAA degradation: first, the root phenotype of ABP1-inactivated plants with elongated cells [16] , reduced root hairs and few or no lateral roots is opposite to the root phenotype of plants with elevated auxin content or roots treated with exogenous auxin [29] , [30] ( Fig. 6a–c ); conversely it is similar to the phenotype of double wei8-1tar mutants that contain reduced auxin [31] . Second, no alteration of free IAA was measured in roots, within up to 2 days following ABP1 inactivation in the immune-modulated SS12K9 line [16] , whereas alterations of gene expression are observed within few hours in similar conditions. Third, as shown above ( Fig. 5c ), the effect of ABP1 inactivation on GA-induced DELLA degradation is similar to the effect of auxin depletion [27] . Fourth, ABP1-inactivated plants exhibit a strong resistance to exogenous auxin with no inhibition of cell elongation and no strong induction of root hair elongation as observed in control roots ( Fig. 6d–g ). And fifth, ABP1 was shown to be required for clathrin-dependent protein internalization and to reduce PIN protein recycling at the plasma membrane [11] , [13] . In consequence, ABP1 inactivation results in endocytosis inhibition, however, without affecting polar localization of PIN auxin efflux proteins [13] , [16] and efficient efflux of auxin was shown to be maintained in roots [16] . More functional PIN efflux carriers at the plasma membrane thus suggest an enhanced ability to transport auxin out of the cells and a predictable decrease in auxin intracellular content. To verify whether the inhibitory effect of ABP1 inactivation on endocytosis is somehow involved in changes of AUX/IAA stability by impairing cellular distribution of auxin, we first mimicked disruption of clathrin-dependent endocytosis by using endocytosis inhibitors and we studied their effects on the stability of AUX/IAAs. Four-day-old Col0 seedlings expressing pHS:AXR3NT-GUS reporter were treated with ikarugamycin or tyrphostin A23 (refs 13 , 32 ), two well-known inhibitors of clathrin-dependent endocytosis, then HS induced as described above. Interestingly, no significant degradation of AXR3NT-GUS was observed within 2 h after HS treatment in the presence of the chemicals, whereas in the same time frame a reduction of 70% was measured for mock-treated roots ( Fig. 7a ). This data indicates that chemical inhibition of endocytosis with either ikarugamycin or tyrphostin A23 promotes a relative stabilization of AXR3NT-GUS, which is potentially resulting from an intracellular decrease in auxin content following inhibition of PIN recycling as predicted. Even more interestingly, this data is opposite to the one resulting from ABP1 inactivation ( Fig. 3 ), whereas both endocytosis inhibitors and ABP1 inactivation impair endocytosis clathrin-dependent [13] , [32] . It clearly indicates that in no way at all the enhanced degradation of AUX/IAA after functional inactivation of ABP1 is originated from endocytosis inhibition. In addition, we took advantage of ABP1conditional plants in rop6-1 and ric1-1 mutants [11] to analyse whether the restoration of endocytosis in roots of these mutants, would be sufficient to restore root growth despite ABP1 knockdown as observed in tir1/afb mutants. Conversely, restoration of endocytosis in roots had no obvious effect on root growth arrest mediated by ABP1 inactivation [16] , indicating that major phenotypic alterations result from a mechanism independent from endocytosis and PIN recycling ( Fig. 7b ). In consequence, the effect of ABP1 on the SCF TIR1/AFB pathway and AUX/IAA stability, which is responsible for the severe developmental defects of ABP1 knockdown, is clearly not mediated by a modulation of protein recycling and hypothesized resulting changes in auxin transport. 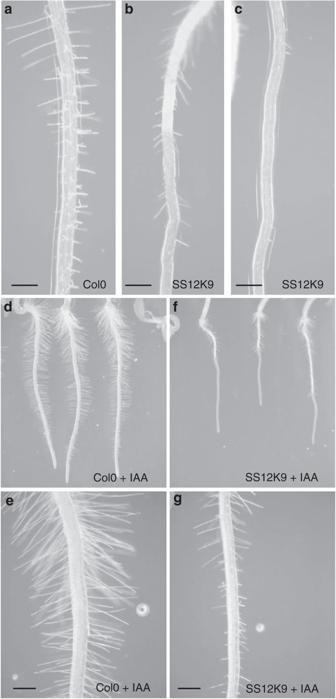Figure 6: Root phenotype and auxin resistance resulting from ABP1 inactivation. (a–c) Roots of ethanol-induced WT (a) and SS12K9 (b,c) grown on vertical plates. Scale bars, 200 μm. (d–g) Primary roots and root hairs of ethanol-induced WT (d,e) and SS12K9 (f,g) grown on vertical plates containing 500 nM IAA for 4 days. Scale bars, 200 μm. Figure 6: Root phenotype and auxin resistance resulting from ABP1 inactivation. ( a – c ) Roots of ethanol-induced WT ( a ) and SS12K9 ( b , c ) grown on vertical plates. Scale bars, 200 μm. ( d – g ) Primary roots and root hairs of ethanol-induced WT ( d , e ) and SS12K9 ( f , g ) grown on vertical plates containing 500 nM IAA for 4 days. Scale bars, 200 μm. 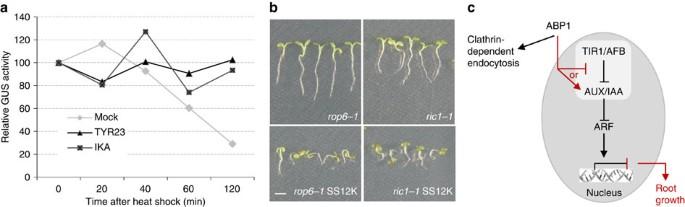Figure 7: ABP1 acts on TIR1/AFB–AUX/IAA pathway independently from endocytosis regulation. (a) Quantification of GUS activity in root samples of WT plants expressingpHS:AXR3NT-GUStreated with tyrphostin A23 (tyr23) or ikarugamycin (ika) clathrin-dependent endocytosis inhibitors. Controls were mock treated. WT seedlings expressing pHS:AXR3NT-GUS were treated with the compounds, then were HS induced for 3 h. Roots were collected immediately after HS treatment for GUS measurement or at the indicated time after HS. (b) Phenotypes of 4-day-old seedlings ofrop6-1andric1-1mutants and SS12K9 into these mutant backgrounds mediating functional inactivation of ABP1; all induced by ethanol since germination. Bar represents 2 mm. (c) Model for ABP1 action on TIR1/AFB–AUX/IAA pathway and for coordination of root growth. ABP1 promotes stabilization of AUX/IAA repressors and maintenance or restoration of transcriptional repression by acting negatively on the TIR1/AFB pathway. Repression of auxin-responsive genes is critical for root growth, especially for cell division and maintenance of the apical meristem that were shown to be under the control of ABP1 (ref.16). Effect of ABP1 on the TIR1/AFB–AUX/IAA pathway does not involve ABP1 control of clathrin-dependent endocytosis. Contributions of the present manuscript are highlighted in red. Full size image Figure 7: ABP1 acts on TIR1/AFB–AUX/IAA pathway independently from endocytosis regulation. ( a ) Quantification of GUS activity in root samples of WT plants expressing pHS:AXR3NT-GUS treated with tyrphostin A23 (tyr23) or ikarugamycin (ika) clathrin-dependent endocytosis inhibitors. Controls were mock treated. WT seedlings expressing pHS:AXR3NT-GUS were treated with the compounds, then were HS induced for 3 h. Roots were collected immediately after HS treatment for GUS measurement or at the indicated time after HS. ( b ) Phenotypes of 4-day-old seedlings of rop6-1 and ric1-1 mutants and SS12K9 into these mutant backgrounds mediating functional inactivation of ABP1; all induced by ethanol since germination. Bar represents 2 mm. ( c ) Model for ABP1 action on TIR1/AFB–AUX/IAA pathway and for coordination of root growth. ABP1 promotes stabilization of AUX/IAA repressors and maintenance or restoration of transcriptional repression by acting negatively on the TIR1/AFB pathway. Repression of auxin-responsive genes is critical for root growth, especially for cell division and maintenance of the apical meristem that were shown to be under the control of ABP1 (ref. 16 ). Effect of ABP1 on the TIR1/AFB–AUX/IAA pathway does not involve ABP1 control of clathrin-dependent endocytosis. Contributions of the present manuscript are highlighted in red. Full size image ABP1 is a long-standing protein that was initially considered to be specifically involved in non-genomic responses to auxin. More recently, accumulating evidence supported that ABP1 is also essential for the control of gene expression in a context-dependent manner [14] , [16] . A reduced auxin effect was reported on the expression of several auxin-responsive genes in roots of plants with impaired ABP1 function [16] ; this apparent reduced responsiveness resulted from a partial derepression following inactivation of ABP1 in the root organ. Genetic and biochemical approaches presented here show that developmental defects observed after ABP1 inactivation are mainly due to altered stability of AUX/IAA repressors and resulting modifications of gene expression. MG132 treatment was efficient in avoiding degradation of AXR3NT-GUS reporter despite inactivation of ABP1, indicating that the 26S proteasome was responsible for the degradation and that AUX/IAA was targeted to degradation by polyubiquitination via involvement of E3 ligases. Genetic data tell us that loss of function in at least two F-boxes among TIR1, AFB2 and AFB3 in ABP1 knockdown restores root growth and AXR3NT-GUS stability. In addition, axr3.1 single mutation affecting the domain of interaction between AXR3 and TIR1/AFBs was sufficient to restore stability. These are strong arguments supporting that ABP1 regulates the stability of AUX/IAAs by controlling somehow their recruitment to SCF TIR1/AFB complexes. We cannot completely rule out that another E3 ligase, presently unknown and distinct from SCF TIR1/AFB , might also contribute to the enhanced degradation of AUX/IAAs in the absence of functional ABP1. Our data show, however, that both ABP1 and TIR1/AFB actions converge on AUX/IAA targets, and act antagonistically to each other. We can conclude that ABP1 is the starting point of a signalling pathway acting as a negative regulator of the SCF TIR1/AFB pathway. Interestingly, the enhanced degradation of AUX/IAA in the absence of functional ABP1 is likely to be independent from the presence of auxin, the SCF TIR1/AFB pathway being constitutively active in the absence of this negative regulation. ABP1 protein is constitutively required to maintain or to restore AUX/IAA-mediated transcriptional repression. An attractive hypothesis is that the ABP1 pathway would confer auxin conditionality to the interaction between TIR1/AFBs and AUX/IAAs. Such conditionality might result from a change in subcellular or nuclei protein localization of AUX/IAA and/or TIR1/AFB proteins [22] , [33] , from the presence or absence of another protein or peptide interacting or competing with one of the component of the transcriptional regulatory module [34] , [35] , [36] , [37] or from post-translational modification affecting the relative affinity between TIR1/AFBs [38] and AUX/IAAs [28] , [39] . A future challenge will be to elucidate the molecular basis of the action of ABP1 on the SCF TIR1/AFB pathway and to identify ABP1 downstream signalling elements filling the gap between ABP1 and the nuclear-localized SCF TIR1/AFB pathway. We showed that modification of endocytosis is not essential for the control of AUX/IAA homeostasis by the ABP1-dependent pathway, thus splitting ABP1 effects into two diverging pathways. Determining whether ROP/RAC GTPases, which were shown to act on endocytosis [11] , [12] , are also part of the ABP1 pathway controlling AUX/IAA stability and gene regulation will be an important question. Interestingly, tobacco and Arabidopsis RAC GTPases were reported to mediate auxin-responsive gene expression [40] and to induce formation of proteolytically active nuclear protein bodies containing AUX/IAA proteins [33] . This would potentially place ROP/RAC GTPases at the node of ABP1 downstream responses. By demonstrating that ABP1 is involved in the control of AUX/IAA homeostasis, we reveal that the SCF TIR1/AFB pathway is far more complex than previously considered, with involvement of a highly regulated and critical balance between stabilization and degradation of transcriptional repressors. Our work provides new basis for exploring positive and negative regulation of auxin signalling and their respective role in the cross-talk with other signalling pathways and coordinated regulation of developmental processes. Plant lines and growth conditions All Arabidopsis genotypes used in this study were in the Columbia (Col0) ecotype, except afb2.1 and afb3.1 that are in the Wassilewskija ecotype [9] . Seeds were germinated under sterile conditions on plates containing 1/2 Murashige and Skoog (MS) basal salt mixture, buffered at pH 5.7 with 2.5 mM 2-( N -morpholino)ethanesulphonic acid, and containing 0.9% vitroagar (Kalys, St Ismier, France). Plates were incubated in a vertical position at 22 °C under constant lighting (99 μmol m −2 s −1 intensity). Ethanol induction of scFv12 expression conferring inactivation of ABP1 was performed as previously described [14] for the indicated time. All reporter constructs and mutations were introgressed into the SS12K9 line by crosses and in each case, homozygous lines were selected before use. Seedling treatments For root growth inhibition assay, seedlings were grown on 1/2 MS mixture containing the indicated concentration of IAA for 4 days, in the presence of ethanol vapours coming from 500 μl of 5% ethanol. For JAZ degradation experiment, 4-day-old seedlings were exposed to 5% ethanol vapours overnight and treated with 200 μM cycloheximide containing 0.1% ethanol. Addition of cycloheximide marks the beginning of the kinetic. Roots were collected at the indicated times after treatments and stored in liquid nitrogen until protein extraction. Treatments with gibberellic acid were performed by immerging overnight ethanol-induced seedlings in 1/2 MS mixture containing 5 μM GA3 for the indicated time. HS induction and GUS activity assay Four-day-old seedlings were ethanol induced overnight before HS treatment was done on plates for 3 h at 37 °C. Drug and mock treatments were applied to the seedlings before HS treatment: 10 μM MG132, 30 μM tyrphostin A23, 30 μM tyrphostin A51 or 5 μM ikarugamycin in 1/2 MS mixture. At the end of the HS treatment, plates were incubated 5 min at 4 °C to stop the HS, except time zero that was collected immediately. β-Glucuronidase (GUS) assays were performed as described in ref. 41 and samples were stained overnight at 37 °C. GUS-stained seedlings were observed without clearing with a MULTIZOOM AZ100 microscope (Nikon Corporation Instruments Company, Japan). Protein extraction was performed in GUS buffer (50 mM NaH 2 PO 4 pH 7, 10 mM EDTA pH8.8, 0.1% Triton X-100, 0.1% Laurylsarcosine and 0.2 mM AEBSF (4-(2-aminoethyl)-benzenesulphonyl fluoride hydrochloride)) without MUG (4 methylumbelliferyl-β- D- glucuronic acid) and total proteins were quantified by Bradford assay. Fluorometric assays were performed by incubating 15 μg total protein in the presence of 2 mM MUG for 2 h in a plate fluorometer (Infinite 200, TECAN) constantly reading fluorescence at 455 nm with an excitation wavelength set at 365 nm. Data were analysed with Excel software (Microsoft) and data were normalized against total protein content. Real-time RT–PCR analysis RNA was extracted from roots of 4-day-old seedlings prior exposure to ethanol vapours and after exposure to ethanol vapours for 8, 24 and 48 h, using a Qiagen RNeasy kit and digested with RNAse-free DNAse on the column following the manufacturer’s instructions (Qiagen S.A., Courtaboeuf, France). First-strand complementary DNAs were synthesized from 5 μg of total RNA using oligo-(dT) 20 and SuperScript III reverse transcriptase according to the manufacturer’s instructions (Life technologies, Invitrogen). Quantitative RT–PCR analyses were performed using Light Cycler FastStart DNA Master Plus SYBR Green I mix (Roche) with specific primers for TIR/AFB as follows: TIR1 forward: 5′-AGA TAA GGG ACT GCC CGT TT-3′, reverse: 5′-GAC CAG CCA CTG TTC GGT AT-3′; AFB1 forward: 5′-ACT GCG AGA ACT GAG GGT GT-3′, reverse: 5′-TCA CAC AGA GAC GGA AGC AC-3′; AFB2 forward: 5′-CGC AGC TGA GAT TCA TGG TA-3′, reverse: 5′-TTG CCT CCA CCG AGT AAA TC-3′; AFB3 forward: 5′-TCG CTG CCA CAT GTA AAG AG-3′, reverse: 5′-TGT GGC TCG AGA ATG CAT AG-3′. Three biological repeats were analysed in duplicate. PCR cycling conditions for amplification were 95 °C for 10 min and then 40–50 cycles of 95 °C for 10 s, 62 °C for 10 s and 72 °C for 15 s followed by 0.1 °C s −1 ramping up to 95 °C for fusion curve characterization. All data were normalized with respect to ACTIN2-8 (ref. 16 ). Protein extraction and western blot analysis Total proteins were extracted from roots of 4 day post-germination seedlings. Samples were grounded in liquid nitrogen and resuspended in preheated denaturing buffer (62.5 mM Tris-HCl pH 6.8, 3% SDS, 10% glycerol, 100 mM dithiothreitol). Samples were heated at 95 °C for 5 min and spun at 5,000 g for 20 min at room temperature to remove cell debris. Protein concentration was estimated by Amidoblack assay. For protein extraction after GA3 treatments, samples were grounded in liquid nitrogen and resuspended in protein extraction buffer (50 mM Tris-HCl pH 7.8, 75 mM NaCl, 15 mM MgCl 2 , 2.5 mM EDTA, 0.1% Nodinet P-40, 1 mM dithiothreitol, 2 mM AEBSF, 0.5 mM NaF, 0.2 mM Na 3 VO 4 , 60 mM β-glycerophosphate, 2 mM MG132, 1 μg ml −1 leupeptine and aprotinin each). Samples were then centrifuged for 30 min at 16,000 g at 4 °C. Supernatants were collected and total proteins were quantified by Bradford assay (Bradford Reagent, Sigma). For scFv12 and ABP1, extraction was performed as previously described [14] . Equal amounts of proteins (20 μg) were mixed with SDS-reducing buffer. Protein sample were separated on 8 or 12% acrylamide (37.5:1) SDS–PAGE, then transferred onto polyvinylidene difluoride membrane (Immobilon-P membrane polyvinylidene difluoride 0.45 μm, Millipore). The membrane was blocked for at least 2 h at room temperature with 5% non-fat dry milk in TBS 0.1% Tween 20 and treated for 1 h with primary antibody at the following dilution: 1/2,000 anti-CUL1 (ref. 20 ), 1/2,500 anti-GFP (BD Biosciences), 1/2,500 anti-HA (Roche), 1/4,000 anti-E-tag and 1/10,000 anti-ABP1 mAb34 (refs 14 , 42 ), in 5% non-fat dry milk in TBS 0.1% Tween 20. For normalization, membranes were reprobed with 1/6,000 anti-TSN primary antibody [43] . Peroxidase activity of horseradish peroxidase-linked secondary antibodies was detected by enzyme-linked chemiluminescence (Immobilon Western HRP substrate, Millipore). Protein expression was quantified by Image J software. All experiments were performed at least in triplicates. How to cite this article: Tromas, A. et al. Auxin-Binding Protein 1 is a negative regulator of the SCF TIR1/AFB pathway. Nat. Commun. 4:2496 doi: 10.1038/ncomms3496 (2013).